Structural insight into the mutual recognition and regulation between Suppressor of Fused and Gli/Ci Hedgehog (Hh) signalling regulates embryonic development and adult tissue homoeostasis. Mutations of its pathway components including Suppressor of Fused (Sufu) and Gli/Ci predispose to cancers and congenital anomalies. The Sufu–Gli protein complex occupies a central position in the vertebrate Hh signalling pathway, especially in mammals. Here structures of full-length human and Drosophila Sufu, the human Sufu–Gli complex, along with normal mode analysis and FRET measurement results, reveal that Sufu alternates between ‘open’ and ‘closed’ conformations. The ‘closed’ form of Sufu is stabilized by Gli binding and inhibited by Hh treatment, whereas the ‘open’ state of Sufu is promoted by Gli-dissociation and Hh signalling. Mutations of critical interface residues disrupt the Sufu–Gli complex and prevent Sufu from repressing Gli-mediated transcription, tethering Gli in the cytoplasm and protecting Gli from the 26S proteasome-mediated degradation. Our study thus provides mechanistic insight into the mutual recognition and regulation between Sufu and Gli/Ci. The Hedgehog (Hh) signal transduction pathway has an essential role in the regulation of embryonic development in both invertebrates and vertebrates, including the patterning of embryonic cuticles and imaginal discs of fruit flies, and the patterning of limbs and neural tubes of chicken, mice and humans [1] . In addition, Hh signalling has also been found to be critical for stem cell maintenance and adult tissue homoeostasis [2] . Mutations of critical components in this pathway such as Patched, Smoothened, Suppressor of Fused (Sufu) and Gli predispose to various types of cancers such as basal cell carcinoma and medulloblastoma [3] , as well as a variety of newborn birth defects such as polydactyly and craniofacial defects [4] . The Hh signalling pathway is mediated mostly by the Gli/Ci family of transcription factors, which comprises three members, Gli1, Gli2 and Gli3 in vertebrates [5] . Gli1 and Gli2 provide most of the transcriptional activator activity, whereas Gli3 contributes to most of the transcriptional repressor activity. Gli1 is also a transcriptional target of Hh signalling and is mutated in human gliomas [6] . In invertebrates such as Drosophila , a single Gli family of protein, Cubitus interruptus (Ci), mediates all aspects of Hh signalling [5] . Sufu is a major regulator of the Gli/Ci transcription factors in both vertebrates and invertebrates [7] , [8] , [9] , [10] , [11] , [12] , [13] and has a more critical role in mammals [14] . Mutations in human Sufu (hSufu) are associated with various kinds of cancers including medulloblastoma (the most frequent malignant paediatric brain tumour) [15] and Gorlin syndrome (also termed naevoid basal cell carcinoma syndrome or basal cell naevus syndrome) [16] . Genetic inactivation of both sufu alleles in mice was embryonic lethal, with a characteristic defect of severely ventralized open neural tube [17] , [18] . Sufu +/− heterozygous mice displayed features of Gorlin syndrome, with 100% penetrance [18] . Sufu inhibits the activity of Gli/Ci both by tethering it in the cytoplasm [7] , [8] , [11] , [12] and by recruiting the SAP18-mSin3-histone deacetylase corepressor complex to Gli-targeted promoters [19] . In addition, Sufu regulates the Gli/Ci protein level by protecting it from being ubiquitinated by the Cul3-Spop (HIB/Roadkill in flies) complex of E3 ubiquitin ligase and being degraded through the 26S proteasome [20] , [21] , [22] , [23] , [24] . Previous studies have revealed that Gli/Ci interacts with Sufu through both its N-terminal [25] , [26] and C-terminal binding sites [27] . The N-terminal Sufu-binding site on Gli/Ci was mapped to the highly conserved ‘SYGHLS’ motif before the five zinc fingers and was found to have a major role in mediating the interaction between Gli/Ci and Sufu [26] . Both Sufu and Gli/Ci proteins are among the most highly conserved components of the Hh signalling pathway. The Sufu–Gli protein complex occupies a central position downstream of the membrane Hh effector Smoothened in the vertebrate Hh signalling pathway, especially in mammals [14] , [28] . Sufu consists of an N-terminal domain (NTD) and a C-terminal domain (CTD) [27] . Although the structure of hSufu-NTD has been reported [27] , a full-length (FL) Sufu structure from any species is still lacking. Moreover, the molecular mechanism of how Sufu employs its two domains to recognize Gli/Ci is controversial [26] , [27] . Here to understand the molecular mechanism of how Sufu recognizes and regulates Gli/Ci, we determined the crystal structures of FL hSufu, FL Drosophila Sufu (dSufu), as well as hSufu in complex with human Gli1 (hGli1). These structures, along with our normal mode analysis, suggest that the conformation of Sufu switches between ‘open’ and ‘closed’ states and is regulated by Gli binding. In addition, our FRET analysis further supports that this conformational switch of Sufu indeed happens in cultured cells and is modulated by Hh signalling. The importance of critical residues on both NTD and CTD of Sufu in recognizing and regulating Gli is further demonstrated by mutagenesis combined with co-immunoprecipitation, subcellular fractionation, immunofluorescence and luciferase assays. Crystal structures of FL hSufu and dSufu Examination of Sufu protein sequences from various organisms by both folding propensity prediction ( Fig. 1a ) and sequence alignment ( Fig. 1b and Supplementary Fig. S1 ) revealed that residues 286–345 of hSufu are intrinsically flexible/unfolded and unconserved, suggesting that these residues might be located in a flexible surface loop with no fixed structure. To facilitate crystallization, we made a couple of hSufu deletion constructs with 20 or 60 internal loop residues, 306–325 or 286–345, deleted (referred to as hSufuΔ20 and hSufuΔ60, respectively; Fig. 1c ). Crystal structures of FL hSufu ( Fig. 1d ), hSufuΔ60 ( Fig. 1e ), hSufuΔ20 ( Fig. 1e ) and FL dSufu ( Fig. 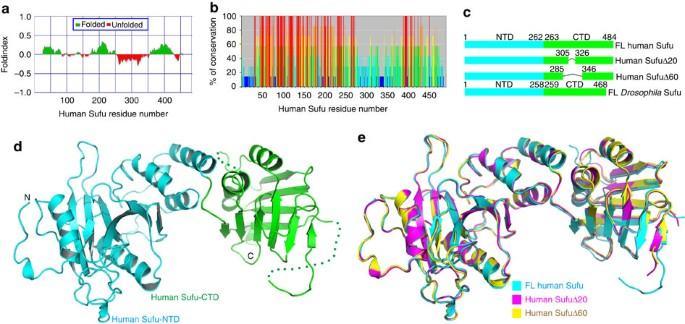Figure 1: Crystal structure of FL human Sufu. (a) Folding propensity of hSufu predicted by the FoldIndex server (http://bip.weizmann.ac.il/fldbin/findex). Green and red denote structured and unstructured regions, respectively. (b) Protein sequences of human, zebrafish, sea urchin, hydra, sponge, mosquito andDrosophilaSufu were aligned by the ClustalW method. Percentage of conservation for each hSufu residue was shown as a red, orange, yellow, green, cyan, light-blue or dark-blue bar from high to low conservation. (c) hSufu and dSufu constructs whose structures were determined in this study. (d) Crystal structure of FL hSufu. Disordered residues with no clear electron density in the structures are denoted by dotted lines. (e) Comparison of crystal structures of FL hSufu, hSufuΔ20 (with deletion of the internal loop residues 306–325) and hSufuΔ60 (with deletion of the internal loop residues 286–345), which are coloured in cyan, magenta and yellow, respectively. The root mean square deviation (RMSD) value is 0.334 Å for 334 aligned Cα atoms between FL hSufu and hSufuΔ20, 0.379 Å for 329 aligned Cα atoms between FL hSufu and hSufuΔ60 and 0.254 Å for 339 aligned Cα atoms between hSufuΔ20 and hSufuΔ60. 2a ) were all subsequently determined to resolutions of 2.25 Å, 3.10 Å, 3.20 Å and 2.70 Å, respectively ( Table 1 ). Structures of FL hSufu and dSufu suggest that they are both monomers and consist of two globular domains, with a short linker (residues 263–267 in hSufu) in between. Sufu-NTD and Sufu-CTD both exhibit α/β folds, with several α helices surrounding a central β sheet ( Figs 1d,e and 2a ). hSufu-NTD in the FL structure is similar to that by itself (PDB code: 1M1L) [27] , with the root mean-square deviation of 0.435 Å for 213 aligned Cα atoms. Figure 1: Crystal structure of FL human Sufu. ( a ) Folding propensity of hSufu predicted by the FoldIndex server ( http://bip.weizmann.ac.il/fldbin/findex ). Green and red denote structured and unstructured regions, respectively. ( b ) Protein sequences of human, zebrafish, sea urchin, hydra, sponge, mosquito and Drosophila Sufu were aligned by the ClustalW method. Percentage of conservation for each hSufu residue was shown as a red, orange, yellow, green, cyan, light-blue or dark-blue bar from high to low conservation. ( c ) hSufu and dSufu constructs whose structures were determined in this study. ( d ) Crystal structure of FL hSufu. Disordered residues with no clear electron density in the structures are denoted by dotted lines. ( e ) Comparison of crystal structures of FL hSufu, hSufuΔ20 (with deletion of the internal loop residues 306–325) and hSufuΔ60 (with deletion of the internal loop residues 286–345), which are coloured in cyan, magenta and yellow, respectively. The root mean square deviation (RMSD) value is 0.334 Å for 334 aligned Cα atoms between FL hSufu and hSufuΔ20, 0.379 Å for 329 aligned Cα atoms between FL hSufu and hSufuΔ60 and 0.254 Å for 339 aligned Cα atoms between hSufuΔ20 and hSufuΔ60. 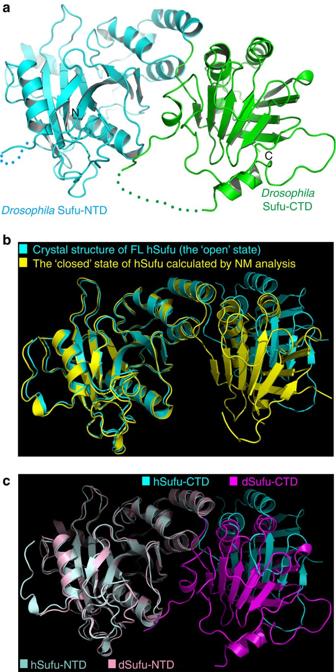Figure 2: There is a breathing motion between the two domains of Sufu proteins. (a) Crystal structures of FL dSufu. Disordered residues with no clear electron density in the structures are denoted by dotted lines. (b) The NM analysis predicts a conformational flexibility of hSufu. The ‘closed’ state of hSufu calculated by the NM analysis was compared with its ‘open’ state (that is, the crystal structure) by superimposing their NTDs. Here we only showed the result from the 7th normal mode (that is, the 1st vibrational mode) of hSufu, which is also described inSupplementary Video 1. The 8th and 9th normal modes (that is, the 2nd and 3rd vibrational modes) of hSufu, both of which also display ‘open’-to-‘closed’ conformational transitions, are described inSupplementary Fig. S3andSupplementary Videos 2 and 3. (c) Structural comparison of hSufu and dSufu, by aligning their NTDs. Full size image Figure 2: There is a breathing motion between the two domains of Sufu proteins. ( a ) Crystal structures of FL dSufu. Disordered residues with no clear electron density in the structures are denoted by dotted lines. ( b ) The NM analysis predicts a conformational flexibility of hSufu. The ‘closed’ state of hSufu calculated by the NM analysis was compared with its ‘open’ state (that is, the crystal structure) by superimposing their NTDs. Here we only showed the result from the 7th normal mode (that is, the 1st vibrational mode) of hSufu, which is also described in Supplementary Video 1 . The 8th and 9th normal modes (that is, the 2nd and 3rd vibrational modes) of hSufu, both of which also display ‘open’-to-‘closed’ conformational transitions, are described in Supplementary Fig. S3 and Supplementary Videos 2 and 3 . ( c ) Structural comparison of hSufu and dSufu, by aligning their NTDs. Full size image Table 1 Data collection and refinement statistics. Full size table There is a breathing motion between the two domains of Sufu hSufu possesses an extended dumb-bell-like shape, with a short linker functioning as a hinge connecting the two globular NTD and CTD domains. Its NTD and CTD pack loosely against each other, with only a few contacts between them ( Supplementary Fig. S2 ). When the intrinsic flexibility of hSufu was analysed by the normal mode (NM) analysis, a breathing motion between the two domains of hSufu was found, resulting in its conformation alternating between a ‘closed and compact’ state and an ‘open and relaxed’ state (that is, the initial crystal structure; Fig. 2b , Supplementary Fig. S3 and Supplementary Movies 1, 2 and 3 ). Strikingly, the FL dSufu structure resembles the predicted ‘closed’ form of hSufu ( Fig. 2c ), and the NM analysis for dSufu also suggests that its conformation switches between ‘closed’ and ‘open’ states ( Supplementary Fig. S4 and Supplementary Movie 4 ). Therefore, both hSufu and dSufu display ‘open’-to-‘closed’ transitions between their NTD and CTD domains, suggesting that this conformational switch is a conserved property of Sufu proteins throughout evolution. When the structure of dSufu was examined, hydrogen bonding interactions between residues of dSufu-NTD (Phe144, Thr146, Asn148, Gly149 and Asp154) and those of dSufu-CTD (Arg309, Ser313 and Gln316) were observed ( Fig. 2a and Supplementary Fig. S5 ). These interactions exist at the far end of dSufu-NTD and -CTD domains, instead of centring around the linker region as in hSufu ( Supplementary Fig. S2 ). Half of these residues (Thr146, Gly149, Ser313 and Gln316) participating in the NTD–CTD interaction in dSufu are not conserved in hSufu ( Supplementary Fig. S1 ), which might be one possible reason accounting for the conformational difference between dSufu and hSufu. On the other hand, we also cannot exclude the possibility that the observed different conformations of hSufu and dSufu are caused by crystal packing effects. Crystal structure of the hSufuΔ60–hGli1 (112–128) complex To understand the structural basis of how Sufu recognizes the Gli/Ci family of transcription factors, we undertook an extensive effort of crystallizing various hSufu or dSufu constructs in complexes with different lengths of Gli1, Gli2, Gli3 or Ci peptides encompassing the Sufu-binding ‘SYGHLS’ motif. We finally succeeded in determining the crystal structure of hSufuΔ60 in complex with human Gli1 (hGli1) (residues 112–128), to the resolution of 1.70 Å ( Table 1 ). Both the Ni 2+ -column pull-down ( Fig. 3a ) and the isothermal titration calorimetry (ITC) assays ( Fig. 3b,c and Table 2 ) demonstrated that hSufuΔ60 bound to hGli1 (97–143) with a similar affinity as FL hSufu, with dissociation constants ( K d ) of 61.3 nM and 95.2 nM, respectively. The sequence of the hGli1 fragment used in the crystallization is highly conserved among Gli/Ci family members ( Fig. 3d ). Therefore, our hSufuΔ60–hGli1 (112–128) complex structure should reflect a general recognition mechanism between Sufu and Gli/Ci proteins. 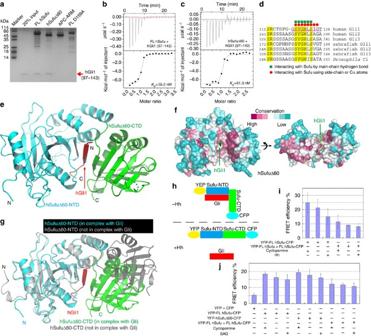Figure 3: The conformation of Sufu is regulated by Gli binding and Hh signalling. (a) hSufuΔ60 interacted with hGli1 (97–143) as strongly as FL hSufu, using the Ni2+-column pull-down assay. (b,c) The dissociation constants (Kd) of FL hSufu and hSufuΔ60 for hGli1 (97–143) were 95.2 nM (b) and 61.3 nM (c), respectively, as measured by the ITC assay. (d) The sequence of the hGli1 (112–128) peptide used for crystallization with hSufuΔ60 is highly conserved among the Gli/Ci family members. The residues with clear electron density in the structure are marked by a magenta underline. (e) Crystal structure of the hSufuΔ60–hGli1 (112–128) complex. (f) hSufu (shown as a surface representation and coloured according to conservation scores) encircles hGli1 (shown as a cartoon representation and coloured in green) using its conserved surface residues. (g) Comparison of structures of hSufuΔ60 by itself and that in complex with hGli1 (112–128) shows that hGli binding stabilizes hSufu in the ‘closed’ conformation. (h) Scheme of our FRET experiment. (i,j) FRET experiments indicate that hSufu tends to be in the ‘open’ form when stimulated by Hh, whereas inhibition of Hh signalling stabilizes hSufu in the ‘closed’ state. Treatment of Hh (i) or the Hh signalling agonist SAG (j) induced a decrease, whereas treatment of the Hh signalling antagonist cyclopamine caused an increase of the FRET signal between YFP and CFP of the YFP–hSufu–CFP fusion protein. As a control, YFP and CFP were separately tagged onto N- and C-terminal ends of hSufu, respectively, and the two constructs were transfected together to see whether there was any FRET signal between NTD and CTD of different hSufu molecules. A higher FRET signal means that the distance between YFP and CFP is closer in space. It is generally considered that the spatial proximity between YFP and CFP is not significant when the measured FRET efficiency is less than or close to 5%. The FRET assay is displayed for each experimental condition (mean±s.d., number of cells examined ≥20). s.d. values are indicated by error bars. Figure 3: The conformation of Sufu is regulated by Gli binding and Hh signalling. ( a ) hSufuΔ60 interacted with hGli1 (97–143) as strongly as FL hSufu, using the Ni 2+ -column pull-down assay. ( b , c ) The dissociation constants ( K d ) of FL hSufu and hSufuΔ60 for hGli1 (97–143) were 95.2 nM ( b ) and 61.3 nM ( c ), respectively, as measured by the ITC assay. ( d ) The sequence of the hGli1 (112–128) peptide used for crystallization with hSufuΔ60 is highly conserved among the Gli/Ci family members. The residues with clear electron density in the structure are marked by a magenta underline. ( e ) Crystal structure of the hSufuΔ60–hGli1 (112–128) complex. ( f ) hSufu (shown as a surface representation and coloured according to conservation scores) encircles hGli1 (shown as a cartoon representation and coloured in green) using its conserved surface residues. ( g ) Comparison of structures of hSufuΔ60 by itself and that in complex with hGli1 (112–128) shows that hGli binding stabilizes hSufu in the ‘closed’ conformation. ( h ) Scheme of our FRET experiment. ( i , j ) FRET experiments indicate that hSufu tends to be in the ‘open’ form when stimulated by Hh, whereas inhibition of Hh signalling stabilizes hSufu in the ‘closed’ state. Treatment of Hh ( i ) or the Hh signalling agonist SAG ( j ) induced a decrease, whereas treatment of the Hh signalling antagonist cyclopamine caused an increase of the FRET signal between YFP and CFP of the YFP–hSufu–CFP fusion protein. As a control, YFP and CFP were separately tagged onto N- and C-terminal ends of hSufu, respectively, and the two constructs were transfected together to see whether there was any FRET signal between NTD and CTD of different hSufu molecules. A higher FRET signal means that the distance between YFP and CFP is closer in space. It is generally considered that the spatial proximity between YFP and CFP is not significant when the measured FRET efficiency is less than or close to 5%. The FRET assay is displayed for each experimental condition (mean±s.d., number of cells examined ≥20). s.d. values are indicated by error bars. Full size image Table 2 Dissociation constants ( K d ) of the interaction between Sufu and Gli proteins. Full size table In the structure, hGli1 (112–128) forms a β-strand and interacts with hSufu by a β-strand addition mechanism [29] . It integrates with β-strands from both hSufu–NTD and hSufu–CTD into a merged β-sheet ( Fig. 3e and Supplementary Fig. S6 ) and is completely encircled by conserved residues of hSufu ( Fig. 3f ). Compared with the ‘open’ conformation of hSufu by itself, association with Gli stabilizes hSufu in the ‘closed’ state by interacting with both domains of it and dragging them together ( Fig. 3g ). To corroborate that the ‘open’-to-‘closed’ conformational change of hSufu indeed happens in vivo , we prepared a YFP–hSufu–CFP construct, in which YFP and CFP were tagged at the N- and C-terminal ends of hSufu, respectively ( Fig. 3h ). When we measured the fluorescence resonance energy transfer (FRET) signal between YFP and CFP of the YFP–hSufu–CFP construct, which was transfected into cultured human embryonic kidney (HEK) 293T cells in the absence or presence of Hh treatment, we found that a lower FRET signal was repetitively measured when stimulated with Hh ( Fig. 3i ) or the Hh signalling agonist SAG ( Fig. 3j and Supplementary Fig. S7 ). In contrast, treatment of cyclopamine, an Hh signalling antagonist, consistently generated a higher FRET signal from YFP–hSufu–CFP ( Fig. 3i,j and Supplementary Fig. S7 ). One possibility to account for the observed FRET signal change is that Hh treatment induces the dissociation of Sufu from Gli [28] , [30] . Without the attachment of Gli, the conformation of Sufu relaxes from ‘closed’ to ‘open’. In the ‘open’ state, Sufu-NTD and Sufu-CTD are further away, hence giving a lower FRET signal. An alternative possibility is that Hh signalling might trigger some post-translational events on Sufu and promotes its conformational switch to the ‘open’ state, thus weakening its association with Gli. Conversely, inhibition of the Hh pathway might stabilize Sufu in the ‘closed’ state, allowing the formation of the Sufu–Gli complex. No matter which of these two possibilities is true, our structural and FRET results suggest that the ‘open’-to-‘closed’ conformational transition of Sufu is correlated with its binding to Gli and is under the regulation of Hh signalling. Key interface residue mutations impair the Sufu–Gli binding Our crystal structure of the hSufuΔ60–hGli1 (112–128) complex reveals that hGli1 engages hSufu through both main-chain and side-chain interactions. The six residues of hGli1, Ser120-Tyr121-Gly122-His123-Leu124-Ser125, form a merged β-sheet with strand β5 from hSufu–NTD and strand β9 from hSufu-CTD ( Fig. 4a ). Moreover, side-chains of hGli1 residues also contribute to the specific recognition with hSufu through both hydrogen bonding and van der Waals interactions. In the center of this interaction network, hGli1–His123 hydrogen bonds with hSufu-Asp159 and hSufu-Tyr147, whereas hGli1-Leu124 forms hydrophobic contacts with hSufu-Leu380, hSufu-Val269 and hSufu-Ala271. At the periphery of the Sufu–Gli interface, hGli1-Ser120 and hGli1-Ser125 hydrogen bond to polar/charged amino acids from hSufu, whereas hGli1-Tyr121, hGli1-Gly122, hGli1-Ile126 and hGli1-Gly127 make hydrophobic interactions with non-polar residues of hSufu ( Fig. 4b ). 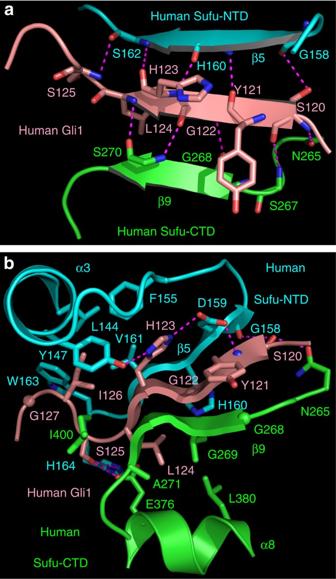Figure 4: The interaction interface between hGli1 and hSufu. (a) The main-chain interactions. (b) The side-chain interactions. hGli1, hSufu-NTD, hSufu-CTD are shown in pink, cyan and green, respectively. Nitrogen and oxygen are coloured in blue and red, respectively. Hydrogen bonds are represented by magenta dashed lines. Figure 4: The interaction interface between hGli1 and hSufu. ( a ) The main-chain interactions. ( b ) The side-chain interactions. hGli1, hSufu-NTD, hSufu-CTD are shown in pink, cyan and green, respectively. Nitrogen and oxygen are coloured in blue and red, respectively. Hydrogen bonds are represented by magenta dashed lines. Full size image Consistent with our structural observations, point mutations of Y147R, D159R, F155A and L380R on hSufu, or their combinations, diminished the binding of hSufu with hGli1 (97–143) by the in vitro Ni 2+ -column pull-down assay ( Fig. 5a ). In addition, quantitative measurement of the binding affinities between various hSufu mutants and hGli1 (97–143) by the ITC assay showed that the double mutant Y147R/F155A of hSufu had a compromised dissociation constant ( K d ) of ~5 μM with hGli1 (97–143) ( Supplementary Fig. S8a and Table 2 ), whereas the Y147R/D159R double mutant ( Supplementary Fig. S8b and Table 2 ), the Y147R/D159R/L380R triple mutant ( Fig. 5b and Table 2 ) and the Y147R/F155A/D159A/L380R ( Supplementary Fig. S8c and Table 2 ) or Y147R/F155A/D159R/L380R ( Supplementary Fig. S8d and Table 2 ) quadruple mutants of hSufu exhibited no detectable binding with hGli1 (97–143). Furthermore, co-immunoprecipitation assays in 293T cells confirmed that mutations of D159R, L380R or Y147R/D159R/L380R in hSufu undermined its recognition of mouse Gli2 (mGli2) (residues 1–633) in vivo ( Fig. 5c ). 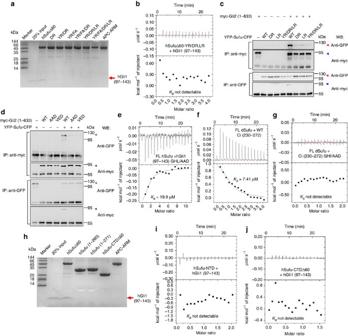Figure 5: Key interface residue mutations on Sufu or Gli/Ci abrogate binding. (a–e) Single or combinations of point mutations of critical residues on Sufu or Gli diminished or abolished their interactions, as revealed by the Ni2+-column pull-down (a), ITC (b,e) and co-immunoprecipitaion assays (c,d). Sufu mutations: D159R (DR), Y147R (YR), F155A (FA) and L380R (LR). Gli mutations: G122A/H123A/L124D in hGli1 or G270A/H271A/L272D in mGli2 (GHL/AAD or AAD), respectively, and G270V/H271E/L272D (VED) in mGli2. Red and blue arrowheads indicate bands of YFP-Sufu-CFP and myc-Gli2, respectively. His-APC-ARM served as a negative control. (f,g) The binding affinity between dSufu and the ‘SYGHIS’ motif of Ci is weaker than that between hSufu and the ‘SYGHLS’ motif of hGli1 (f) and triple mutation of G257A/H258A/I259D (GHI/AAD) in Ci (230–272) eliminated its interaction with dSufu (g). (h–j) Sufu-NTD or Sufu-CTD alone is insufficient to bind to hGli1 (97–143), as shown by the Ni2+-column pull-down (h) and ITC assays (i,j). Figure 5: Key interface residue mutations on Sufu or Gli/Ci abrogate binding. ( a – e ) Single or combinations of point mutations of critical residues on Sufu or Gli diminished or abolished their interactions, as revealed by the Ni 2+ -column pull-down ( a ), ITC ( b , e ) and co-immunoprecipitaion assays ( c , d ). Sufu mutations: D159R (DR), Y147R (YR), F155A (FA) and L380R (LR). Gli mutations: G122A/H123A/L124D in hGli1 or G270A/H271A/L272D in mGli2 (GHL/AAD or AAD), respectively, and G270V/H271E/L272D (VED) in mGli2. Red and blue arrowheads indicate bands of YFP-Sufu-CFP and myc-Gli2, respectively. His-APC-ARM served as a negative control. ( f , g ) The binding affinity between dSufu and the ‘SYGHIS’ motif of Ci is weaker than that between hSufu and the ‘SYGHLS’ motif of hGli1 ( f ) and triple mutation of G257A/H258A/I259D (GHI/AAD) in Ci (230–272) eliminated its interaction with dSufu ( g ). ( h – j ) Sufu-NTD or Sufu-CTD alone is insufficient to bind to hGli1 (97–143), as shown by the Ni 2+ -column pull-down ( h ) and ITC assays ( i , j ). Full size image Gly122, His123 and Leu124 of hGli1 are in the center of the hSufu–hGli1 interface. Triple mutations of the corresponding residues in mGli2 (1–633), G270A/H271A/L272D or G270V/H271E/L272D weakened its interaction with hSufu in the co-immunoprecipitation assay in 293T cells ( Fig. 5d ). Furthermore, triple mutations of these three residues to Ala/Ala/Asp in hGli1 (97–143) attenuated its binding affinity for FL hSufu and hSufuΔ60 in the ITC assay, with K d values of 10–20 μM ( Fig. 5e , Supplementary Fig. S9 and Table 2 ). In the case of the Drosophila dSufu–Ci complex, the binding affinity of wild-type (WT) Ci (230–272) for dSufu is weaker than that of hGli1 (97–143) for hSufu ( Fig. 5f and Table 2 ), thus triple mutation of G257A/H258A/I259D in Ci (230–272) eliminated its binding with dSufu ( Fig. 5g and Table 2 ). As our results demonstrate that the highly conserved ‘SYGHLS’ motif of Gli/Ci proteins is critical for their association with Sufu, a natural question is whether other proteins containing this motif also interact with Sufu. We performed a BLAST search on the human protein sequence database and indeed found some proteins possessing sequences identical or similar to the ‘SYGHLS’ motif ( Supplementary Table S1 ). However, possession of the ‘SYGHLS’ motif might not automatically guarantee a stable association with Sufu ( Supplementary Note 1 , Supplementary Fig. S10 ). The local protein structural environment where this motif resides is also very important for its recognition by Sufu as well. Sufu-NTD/CTD alone do not stably bind to Gli’s SYGHLS motif Our crystal structure shows that the hGli1 peptide is sandwiched between the NTD and CTD of hSufu, and both domains of hSufu contribute to the recognition of hGli1. In agreement with this structural observation, our Ni 2+ -column pull-down ( Fig. 5h ) and ITC ( Fig. 5i,j and Table 2 ) assays demonstrated that hSufu-NTD or hSufu-CTD alone was not sufficient for stable complex formation with hGli1 (97–143), consistent with the previous report that IVS8+1G→A, a frameshift mutation of hSufu found in both medulloblastoma and Gorlin syndrome patients that resulted in a truncated form of hSufu-Δex8 (residues 1–322, instead of WT hSufu residues 1–484), and hSufu (residues 212–484) were unable to bind to Gli2 and anchor it in the cytoplasm [15] , [16] . Despite considerable effort, we only succeeded in crystallizing hSufuΔ60 in complex with a 17-amino acid peptide of hGli1 encompassing residues 112–128. Although this peptide still interacted with both FL hSufu and hSufuΔ60, its binding affinity for hSufu was 20–60 times weaker than that of hGli1 (97–143) ( Table 2 and Supplementary Fig. S11a,b ). Interestingly, a 27-residue peptide of hGli1 (107–133) displays a dissociation constant in between ( Table 2 and Supplementary Fig. S11c ), and a 37-residue peptide hGli1 (102–138) associates with hSufu with almost the same affinity as hGli1 (97–143) ( Table 2 and Supplementary Fig. S11d ). These data exhibited a progressively strengthening interaction with hSufu with the increasing length of hGli1 peptides, and suggested that additional interactions beyond residues 112–128 possibly exist between the N-terminal part of hGli1 and hSufu. Key residue mutations compromise regulation of Gli by Sufu Sufu is a major regulator of the Gli/Ci transcription factors, especially in mammals [14] . Among the three Gli family members, Gli1 is a transcriptional activator and efficiently promotes its target gene transcription in luciferase assays [7] , [9] , [19] , [23] , [26] , [27] . Moreover, unlike Gli2 and Gli3, Gli1 does not associate with Spop [23] and the protein expression level of Gli1 has not been found to be regulated by Spop and Sufu [20] , [22] , [23] , [24] , which would simplify the assay results. Therefore, we selected Gli1 to examine how various mutations on Sufu or Gli affect the regulation of Gli-mediated transcription by Sufu. When WT hSufu was co-transfected together with hGli1, it effectively repressed the hGli1-mediated transcription ( Fig. 6a ). On the other hand, Sufu point mutants of D159R, L380R or Y147R/D159R/L380R were unable to suppress the transcription promoted by hGli1 ( Fig. 6a ). In addition, point mutations or deletions of residues Gly122, His123 and Leu124 in hGli1 made it no longer under the regulation of hSufu ( Fig. 6b ). 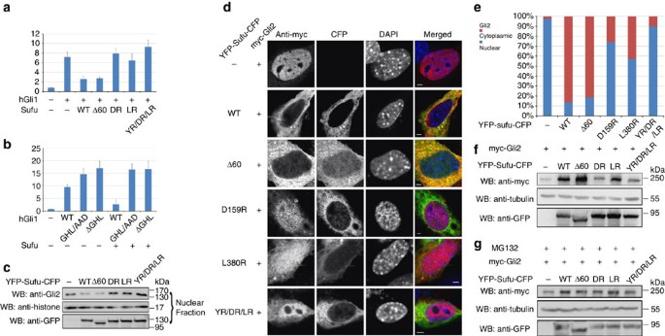Figure 6: Mutation or deletion of key interface residues abolishes the regulation of Gli by Sufu. (a,b) Point mutations or deletion of important interface residues on Sufu (a) or Gli1 (b) attenuated the inhibition of the Gli1-mediated transcription by Sufu. The luciferase assay is displayed for each experimental condition (mean±s.d., number of repeats=3). s.d. values are indicated by error bars. (c–e) Point mutations of crucial residues on Sufu mediating Gli binding subverted its function of anchoring Gli2 in the cytoplasm and preventing Gli2 from translocating to the nucleus, as demonstrated by the fractionation assay to examine endogenous Gli2 (c) and the immunofluorescence assay to examine exogenously transfected Gli2 (d). In the merged images of immunofluorescence experiments, red, green and blue colours represent anti-myc, CFP and DAPI staining, respectively. The scale bars represent 2 μm. (e) Quantitation of the results inFig. 6d. The percentages of Gli2 in the cytoplasm and the nucleus when co-transfected with different Sufu constructs are shown. (f,g) In contrast to WT Sufu, point mutants of Sufu with critical Gli-binding residues altered were not able to protect Gli from the 26S proteasome-mediated degradation. (f) Sufu point mutants unable to bind to Gli were also not able to stabilize Gli2. Sufu mutations: Y147R (YR), D159R (DR) and L380R (LR). (g) When treated by the 26S proteasome inhibitor MG132, cells expressing the same Sufu mutants as in (f) had the same Gli2 protein expression levels as those expressing WT Sufu. Figure 6: Mutation or deletion of key interface residues abolishes the regulation of Gli by Sufu. ( a , b ) Point mutations or deletion of important interface residues on Sufu ( a ) or Gli1 ( b ) attenuated the inhibition of the Gli1-mediated transcription by Sufu. The luciferase assay is displayed for each experimental condition (mean±s.d., number of repeats=3). s.d. values are indicated by error bars. ( c – e ) Point mutations of crucial residues on Sufu mediating Gli binding subverted its function of anchoring Gli2 in the cytoplasm and preventing Gli2 from translocating to the nucleus, as demonstrated by the fractionation assay to examine endogenous Gli2 ( c ) and the immunofluorescence assay to examine exogenously transfected Gli2 ( d ). In the merged images of immunofluorescence experiments, red, green and blue colours represent anti-myc, CFP and DAPI staining, respectively. The scale bars represent 2 μm. ( e ) Quantitation of the results in Fig. 6d . The percentages of Gli2 in the cytoplasm and the nucleus when co-transfected with different Sufu constructs are shown. ( f , g ) In contrast to WT Sufu, point mutants of Sufu with critical Gli-binding residues altered were not able to protect Gli from the 26S proteasome-mediated degradation. ( f ) Sufu point mutants unable to bind to Gli were also not able to stabilize Gli2. Sufu mutations: Y147R (YR), D159R (DR) and L380R (LR). ( g ) When treated by the 26S proteasome inhibitor MG132, cells expressing the same Sufu mutants as in ( f ) had the same Gli2 protein expression levels as those expressing WT Sufu. Full size image WT hSufu and hSufuΔ60 anchor the FL Gli2 protein in the cytoplasm and prevent it from translocating to the nucleus ( Fig. 6c,d,e ), as reported previously [7] , [8] , [11] , [12] . In contrast, single point mutants of D159R or L380R or the triple mutant Y147R/D159R/L380R of hSufu could not tether endogenously or exogenously transfected FL Gli2 in the cytoplasm, which appeared in the nucleus ( Fig. 6c,d,e ). These cell biological assay results provide a further corroboration on our biochemical observations that point mutations of key interface residues on Sufu impaired its complex formation with Gli. Sufu not only negatively regulates the activity of Gli, but also protects its protein expression level from being downregulated by the Spop-mediated ubiquitination and degradation [20] , [21] , [22] , [23] , [24] . Indeed, mGli2 was stabilized by WT hSufu or hSufuΔ60 ( Fig. 6f ). In contrast, the D159R, L380R or Y147R/D159R/L380R point mutants of hSufu were not able to maintain the same protein level of exogenously transfected mGli2 ( Fig. 6f ). When the 26S proteasome inhibitor MG132 was added in this experiment, the protein levels of mGli2 became the same for all the hSufu mutants as for WT hSufu and hSufuΔ60 ( Fig. 6g ). These results suggest that point mutations of Y147R/D159R/L380R on hSufu impaired its ability to counteract the 26S proteasome-mediated protein degradation of Gli, presumably because of defective Gli binding caused by these mutations. Sufu is a crucial regulator of the Gli/Ci family of transcription factors in both vertebrates and invertebrates, and the Sufu–Gli protein complex forms the core of the vertebrate Hh signalling pathway downstream of Smoothened [28] . Our crystal structures of FL hSufu, FL dSufu and the hSufuΔ60-hGli1 (112–128) complex, as well as our normal mode analysis, reveal that the Sufu protein possesses an intrinsic conformational flexibility, with the arrangement of its NTD and CTD domains alternating between ‘open’ and ‘closed’ states. Binding to Gli stabilizes Sufu in the ‘closed’ state ( Fig. 3e ), with the β-strand of Gli acting as a ‘glue’ to bring strands β5 of Sufu-NTD and β9 of Sufu-CTD together. In response to Hh, the conformation of Sufu relaxes to the ‘open’ state ( Fig. 3h,i,j ) and it is dissociated from Gli [28] , [30] . Therefore, the ‘closed’ state of Sufu is favored when it is associated with Gli and when the Hh signal is absent, and the ‘open’ conformation of Sufu prevails when it dissociates from Gli and is promoted by Hh signalling. The Sufu-binding fragment of Gli/Ci, the ‘SYGHLS’ motif, is completely surrounded by conserved residues from Sufu ( Fig. 3f ). It was reported that two of the major HIB-binding sites on Ci are at residues 216–227 and 368–376, which are nearby its ‘SYGHIS’ motif, residues 255–260 (ref. 22 ). In the case of Gli3, it is only known that its N-terminal region (residues 242–477 of mouse Gli3) contains a Spop-binding site, but its exact location has not been pinpointed [24] . It is likely that the complex formation between Sufu and Gli/Ci creates a steric hindrance for Spop/HIB, thus prohibiting the Spop/HIB-mediated ubiquitination and degradation of Gli/Ci. Moreover, Spop/HIB has been reported to form a dimer and make multivalent interactions with Gli/Ci [22] , therefore the complex formation between Sufu and Gli/Ci would indeed leave barely enough space for a Spop/HIB dimer to occupy two adjacent binding sites on Gli/Ci at the same time. It would be worthwhile to investigate further the underlying mechanism(s) of how Sufu inhibits Gli/Ci degradation, which could be Spop/HIB-dependent or -independent. Previous investigations on the molecular mechanism of interaction between Sufu and Gli/Ci have obtained somewhat contradictory results [26] , [27] . Part of the reason might be that Sufu uses both its NTD and CTD to clamp Gli/Ci in the middle, hence any attempt using the deletion mapping approach might be hampered by the pitfall of damaging the structural integrity of FL Sufu and thus yield misleading results. Studies conducted by mutation-based approaches also need to be carefully evaluated so as not to be over-interpreted. For example, the highly conserved ‘HGRHFTYK’ motif (residues 391–398 in hSufu) is reported to be required for stable interaction with Gli/Ci, and mutation of this motif disrupted the binding and inhibition of Gli by Sufu [27] . However, our structure of the hSufu–hGli1 complex shows that these residues are not in direct contact with Gli ( Fig. 3e ). This fragment forms strand β13 of hSufu–CTD ( Fig. 1c ) and juxtaposes strand β9, which engages hGli1 by β-sheet interaction ( Fig. 4a and Supplementary Fig. S12 ). Mutation of the ‘HGRHFTYK’ motif to alanines would potentially affect the structural integrity of β13, which would in turn obstruct the formation of β9 and even the entire Sufu–CTD. Without the participation of Sufu-CTD, especially that of β9, a stable complex between Sufu and the ‘SYGHLS’ motif of Gli would not be achieved. Our ITC and Ni 2+ column pull-down results suggested that the NTD or CTD of Sufu alone was not sufficient for stable complex formation with the ‘SYGHLS’ motif of Gli/Ci ( Fig. 5h,i,j ). However, it was also reported that Sufu-NTD and -CTD had reduced but detectable interactions with FL Gli1 and Sufu-NTD was sufficient for the inhibition of Gli1- and Gli2-dependent transcriptional activation [31] . Gli/Ci proteins contain a second Sufu-binding site in their C-terminal halves [27] , but its precise location has not been pinpointed. Determination of the exact position of this C-terminal Sufu-binding site on Gli/Ci and elucidation of its role in the regulation of Gli/Ci by Sufu deserve further attention. In vertebrates, especially in mammals, primary cilium has an important role in Hh signalling. Many key Hh signalling components such as Patched and Smoothened are localized to primary cilia and their ciliary localizations are regulated by Hh [32] . Sufu translocates to cilia coordinately with Gli and its ciliary localization depends on Gli [28] , [33] . The regulation of Gli by Sufu is independent of cilia [23] , [34] , but the Hh/Smo-induced release of Sufu from Gli requires cilia [28] , [34] . It is conceivable that in response to Hh, some kind of cilia-specific post-translational modification event such as phosphorylation happens on Gli or Sufu, resulting in the dissociation of Gli from Sufu in cilia and the subsequent translocation of Gli to the nucleus. Intriguingly, there are many potential phosphorylation sites within and surrounding the Sufu-binding ‘SYGHLS’ motif in Gli/Ci. It might be warranted to investigate whether any Hh-induced and cilia-dependent phosphorylation occurs on Gli or Sufu and whether there exists any cilia-localized kinase specifically mediating these phosphorylation events. Mutations of the human Sufu gene predispose individuals to cancers. The tumour suppressor function of Sufu is considered mainly as working through restraining the activities of the Gli transcription factors, whose mutations are also correlated with tumours and congenital malformations. Understanding the complex interplay between Sufu and Gli at the structural level would deepen our understanding of the molecular mechanism of how pathogenic mutations of Sufu and Gli work. For example, a frameshift mutation IVS8+1G→A was found in both medulloblastoma and Gorlin syndrome patients [15] , [16] . This mutation resulted in a truncated Sufu-Δex8 protein (residues 1–322, instead of WT hSufu residues 1–484), in which the majority of the CTD domain of hSufu was removed ( Supplementary Fig. S1 ). This result is fully consistent with our finding that Sufu-CTD is indispensible in the recognition and regulation of Gli proteins. The Gli transcription factor represents a potential therapeutic target, and understanding of the Sufu–Gli protein complex might also inspire the development of pharmaceutical approaches to rein in aberrant activities of Gli in cancers. Protein expression and purification The cDNA encoding FL hSufu and dSufu were cloned into the pFastBac-HTB or HTA vector with N-terminal His-tags. Recombinant bacmids were produced from DH10Bac cells and were used to transfect Sf9 cells to make the baculovirus, which was then used to infect High Five suspension insect cells (Invitrogen). After three cycles of freezing and thawing, the cell lysates were centrifuged and first purified by the Ni 2+ -NTA affinity chromatography (Qiagen), with the binding buffer containing 25 mM Tris (pH 8.0), 300 mM sodium chloride and 20 mM imidazole, and the elution buffer containing 25 mM Tris (pH 8.0), 300 mM sodium chloride and 500 mM imidazole. The eluted fractions was further purified by the Source 15Q anion exchange chromatography (GE healthcare), equilibrated with buffer A containing 25 mM Tris (pH 8.0) and 2 mM dithiothreitol eluted with buffer A plus a linear sodium chloride concentration gradient of 0–500 mM. FL hSufu was treated with the TEV protease at 4 °C to cleave the His-tag, whereas FL dSufu was not. hSufuΔ60 (with 60 internal loop residues 286–345 deleted) and hSufuΔ20 (with 20 internal loop residues 306–325 deleted) were cloned into the pET28a vector (Novagen), both with N-terminal His-tags. Both deletion constructs were expressed in the E. coli strain BL21(DE3) at 18 °C. After sonication and centrifugation, the supernatant of cell lysates was purified by the Ni 2+ -NTA affinity chromatography (Qiagen). All the proteins (FL hSufu, hSufuΔ60, hSufuΔ20 and FL dSufu) were further purified by the Superdex200 gel filtration chromatography (GE Healthcare). The Superdex200 buffer contained 10 mM Tris–HCl (pH 8.0), 100 mM sodium chloride, 5 mM dithiothreitol and 1 mM EDTA. Peak fractions were combined and concentrated to 10 mg ml −1 for crystallization experiments. Two hSufu-NTD constructs (residues 1–260 or 1–271) and one hSufu-CTD construct (residues 252–484 with internal loop residues 286–345 deleted) were similarly cloned into the pET28a vector. Various point mutations on the FL hSufu or hSufuΔ60 background (double mutants Y147R/F155A and Y147R/D159R, triple mutant Y147R/D159R/L380R and quadruple mutants Y147R/F155A/D159A/L380R and Y147R/F155A/D159R/L380R) were introduced by the whole-plasmid PCR and Dpn I digestion method and identities of individual clones were verified by sequencing. All the mutant Sufu proteins were purified using the same procedure as for the WT protein. All the constructs used for experiments in cultured cells were cloned into the pcDNA3.1 vector. hSufu constructs were tagged with YFP at their N termini and with CFP at their C termini, or only with YFP at the N termini or only with CFP at the C termini. Gli constructs were tagged with myc at their N termini. Mutations were introduced using the whole-plasmid PCR and Dpn I digestion method. Peptide synthesis Peptides of hGli1 (112–128), hGli1 (107–133), hGli1 (102–138), WT or the G122A/H123A/L124D triple mutant of hGli1 (97–143) and WT or the G257A/H258A/I259D triple mutant of Drosophila Ci (230–272) were synthesized chemically. All the synthesized peptides were purified to 95% purity by reverse-phase HPLC (Scilight Biotechnology LLC). Crystallization and structure determination All the crystallization experiments were performed by the hanging-drop vapor-diffusion method. The lysine methylation method [35] was used to improve the diffraction quality of hSufuΔ60 crystals. Crystals of lysine-methylated hSufuΔ60 were grown at 14 °C, with the reservoir solution containing 8% PEG 3,350 and 0.15 M ammonium tartrate. Crystals were transferred to the crystallization buffer supplemented with 60% sodium malonate before being flash-frozen. An X-ray diffraction data set of hSufuΔ60 at 2.25 Å was collected at the beamline BL17U1 at Shanghai Synchrotron Radiation Facility (SSRF, China), using an ADSC Quantum 315r CCD area detector. The diffraction data were processed using the HKL2000 software [36] . The crystal was in space group C 222 1 and contained one molecule in each asymmetric unit. The structure of hSufuΔ60 was solved by the molecular replacement method with the CCP4 programme Phaser [37] , [38] , using the hSufu-NTD structure (PDB code: 1M1L) [27] as the searching model. The remaining model was built manually with Coot [39] . After refinement by the CCP4 programme REFMAC [37] , [40] , the final model includes residues 1–6, 22–279, 362–450 and 457–481 of hSufu, with Lys57 methylated. Crystals of hSufuΔ20 were grown at 14 °C, with the reservoir solution containing 16% PEG 3,350 and 0.1 M ammonium tartrate. Crystals were serially transferred from the crystallization drop to the crystallization buffer supplemented with 10%, 20% and 25% glycerol for 5 min each to dehydrate before being frozen. One data set of hSufuΔ20 at 3.1 Å was collected at the SSRF beamline BL17U1. The crystal was in space group C 2 and contained two molecules in each asymmetric unit. The structure was solved by the CCP4 programme Phaser [37] , [38] , using the structure of hSufuΔ60 as the searching model. After refinement by the CCP4 programme REFMAC [37] , [40] , the final model contains hSufu residues 1–3, 20–279, 362–450 and 455–481 in one molecule and residues 1–5, 20–280, 361–450 and 456–481 in the other molecule. Crystals of FL hSufu were initially grown at 14 °C as twinned thin plates, with the reservoir solution containing 20% PEG 3,350 and 0.2 M potassium chloride. To obtain single crystals, the original crystals were crushed and used for microseeding at 8 °C. Crystals were transferred to the crystallization buffer supplemented with 60% sodium malonate before being flash-frozen. One data set of hSufu at 3.2 Å was collected at the SSRF beamline BL17U1. The crystal was in space group C 222 1 and contained one molecule in each asymmetric unit. The structure was solved by Phaser [37] , [38] , using the structure of hSufuΔ60 as the searching model. After refinement by the CCP4 programme REFMAC [37] , [40] , the final model includes hSufu residues 21–280, 356–452 and 457–481. Crystals of FL dSufu were initially obtained at 8 °C as twinned thin plates using the hanging-drop vapor-diffusion method, with the reservoir solution containing 20% PEG 3,350 and 0.2 M magnesium acetate. To obtain single crystals, the original crystals were crushed and used for microseeding in the reservoir solution containing 16% PEG 3,350 and 0.16 M magnesium acetate at 4 °C. Crystals were transferred to the crystallization buffer supplemented with 60% sodium malonate before being flash-frozen. One data set of FL dSufu at 2.7 Å was collected at the SSRF beamline BL17U1. The crystal was in space group C 222 1 and contained one molecule in each asymmetric unit. The structure was solved using the molecular replacement method by Phaser [37] , [38] , using the structure of hSufu-NTD (residues 22–260) and hSufu-CTD (residues 267–481) as searching models. The refinement was performed by the CCP4 programme REFMAC [37] , [40] . The final refined model includes residues 1–3, 13–296 and 308–454 of dSufu. The hSufuΔ60 protein was mixed with the hGli1 (112–128) peptide at 1:1.5 molar ratio and used for crystallization screening. Crystals were grown at 4 °C or 14 °C using the hanging-drop vapor-diffusion method, with the reservoir solution containing 20% PEG 3,350 and 0.2 M magnesium chloride. Crystals were transferred to the crystallization buffer supplemented with 25% glycerol before being flash-frozen. One diffraction data set at 1.7 Å was collected at the beamline BL17U1 at SSRF. The crystal was in space group C 222 1 and contained one molecule in each asymmetric unit. The crystal structure was solved using the molecular replacement method with the CCP4 programme Phaser [37] , [38] , using the structures of hSufu-NTD (residues 22–260) and hSufu-CTD (residues 267–481) as searching models. The refinement was performed by the CCP4 programme REFMAC [37] , [40] . The final model includes residues 28–278, 359–450 and 457–480 of hSufu and residues 119–128 of hGli1. The qualities of all the structures determined were checked with the CCP4 programme PROCHECK [37] , which shows a good stereochemistry according to the Ramachandran plot. NM analysis The structural coordinates of FL hSufu and FL dSufu were submitted for the NM analysis using the Elastic Network Model server ( http://www.igs.cnrs-mrs.fr/elnemo/ ) [41] , which is a fast and simple tool to compute the low-frequency normal modes of a protein. The following parameters were used for the calculation: NMODES=5, DQMIN=−300, DQMAX=300 and DQSTEP=20. The major vibrational modes generated by the server were used for further analysis. According to the Analytical Mechanics theory of physics, the number of total normal modes of the protein system under examination would be 3 N — M , with N being the number of atoms in the protein system and M being the number of constraints imposed on the system (such as bond lengths, bond angles, dihedral angels, and so on). Among these 3 N — M normal modes, three of them are translational modes of the system as a whole and another three are rotational modes of the system as a whole. The rest of the normal modes, which consists of 3 N — M —6 modes, are all vibrational modes. In the output of the normal mode analysis server, the calculated normal modes are listed according to their importance (the one slower in vibrational frequency is considered as more important). The 7th normal mode in this list, which is the 1st vibrational mode (the first six normal modes are translational and rotational modes of the system as a whole), is the one slowest in vibrational frequency and thus is regarded as the most important vibrational mode. The 8th normal mode in this list, which is the 2nd vibrational mode, is the one second slowest in vibrational frequency and is regarded as the second most important vibrational mode, and so on. As the total numbers of vibrational modes of our systems are too many, we only selected the most major ones (the 7th, 8th and 9th normal modes of FL hSufu and the 7th normal mode of dSufu) for further analysis. Molecular graphics All protein structure figures were generated by the PyMOL programme ( http://www.pymol.org ). Sequence conservation of hSufu mapped onto the surface of its crystal structure was generated by the ConSurf server ( http://consurf.tau.ac.il ) [42] . Ni 2+ column pull-down assay Binding assays between purified His-tagged WT or various mutant hSufu proteins and the WT hGli1 (97–143) peptide were performed by the Ni 2+ column pull-down assay according to standard procedures [43] . The Gli peptide was added to pre-immobilized His-hSufu protein on the Ni 2+ -NTA affinity column (Qiagen) at 4 °C, washed with the Ni 2+ column binding buffer (25 mM Tris (pH 8.0), 300 mM NaCl and 20 mM imidazole (pH 8.0)) and eluted with the Ni 2+ column elution buffer (25 mM Tris (pH 8.0), 300 mM NaCl and 500 mM imidazole (pH 8.0)). Samples from the input hGli1 peptide solution and various eluted protein fractions were analysed by SDS–PAGE and Coomassie Blue staining. Isothermal titration calorimetry (ITC) assay ITC experiments were performed using an ITC200 system (MicroCal) at 25 °C. The buffer contained 25 mM HEPES-Na, (pH 7.4) and 100 mM NaCl. Proteins were centrifuged and degassed before the experiment. Typically, a 200 μM WT or point-mutant FL hSufu, hSufuΔ60 or FL dSufu protein was injected 16 times in 2.5 μl aliquots (or 20 times in 2.0 μl aliquots) into a 200-μl sample cell containing hGli1 (112–128), hGli1 (107–133), hGli1 (102–138), WT or point mutant hGli1 (97–143) and WT or point mutant Drosophila Ci (230–272) peptide at a concentration of 20 μM. Data were fit with a nonlinear least-square routine using a single-site binding model with Origin for ITC version 7.0 (MicroCal), varying the stoichiometry ( n ), the enthalpy of the reaction (Δ H ) and the association constant ( K a ). Cell culture and transfection Human embryonic kidney (HEK) 293T cells and NIH-3T3 cells were cultured in Dulbecco’s modified Eagle’s medium (HyClone) and transfected with Lipofectamine 2000 (Invitrogen) under standard protocols. Cells were harvested 48 h after transfection. Antibodies Primary antibodies used in this study were mouse anti-GFP (Santa Cruz), mouse anti-myc (Sigma), mouse anti-β-tubulin (DSHB), rabbit anti-histone and rabbit anti-Gli2 (Abcam). Secondary antibodies were purchased from Millipore. Antibody dilution ratios used for western blotting are all 1:1,000. Subcellular fractionation Nuclear and cytoplasmic extracts were isolated by subcellular fractionation using the NE-PER kit (Pierce) according to the manufacturer’s instruction. Immunoprecipitation and western blot analysis HEK293T cells were lysed by the lysis buffer (50 mM Tris–HCl (pH 8.0), 0.1 M NaCl, 10 mM sodium fluoride, 1 mM sodium vanadate, 1% NP-40, 10% glycerol and 1.5 mM EDTA, supplemented with the protease inhibitor cocktail) for 30 min at 4 °C. After centrifugation, cell lysates were incubated with 2 μg of indicated antibodies for at least 2 h, then combined with 30 μl Protein A/G PLUS agarose (Santa Cruz) and incubated for 1 h at 4 °C. Beads were washed with 1 ml of lysis buffer for three times. Uncropped scans of western blots are shown in Supplementary Fig. S13 . Luciferase assay NIH-3T3 cells cultured in 24-well plate were co-transfected with 250 ng of 8 × GLIBS-luciferase reporter, 5 ng of Renilla plasmids and 500 ng of indicated constructs. After transfection for 48 h, dual-luciferase measurements were performed using the Dual-GloTM luciferase assay system (Promega). Luminescence was measured as relative light units (RLU). Statistical significance was determined using the Student’s t -test. Immunofluorescence NIH-3T3 cells were plated in 24-well plates and fixed in 4% formaldehyde for 10 min. Cells were permeabilized with phosphate-buffered saline (PBS) with 0.25% Triton X-100 for 3 min. Non-specific binding sites were blocked with 2% BSA in the PBST buffer (PBS containing 0.5% Tween-20). Cells were stained with primary antibodies diluted in PBST with 1% BSA for 1 h at room temperature. After washing for three times in PBST, cells were incubated for 1 h with appropriate secondary antibodies and 1 μg ml −1 of 4',6-diamidino-2-phenylindole (DAPI) for nuclear staining in PBST with 1% BSA. Images were taken using the Leica LAS SP5 confocal microscope. Quantitation was based on >50 cells. Statistical significance was determined using the Student’s t -test ( Fig. 6e ). Fluorescence resonance energy transfer (FRET) analysis The FRET experiment was performed as previously described [44] , [45] . Briefly, HEK293T cells were transfected with indicated constructs. Cells were fixed in 4% formaldehyde for 10 min. Fluorescence signals were acquired with the Leica TCS SP5 Confocal microscope DM6000 (for Fig. 3i ) or DMI6000 (for Fig. 3j ). CFP signal was obtained once before photobleaching and once after photobleaching YFP at the top half of each cell, leaving the bottom half of each cell as the internal control. Each data set was based on >20 individual cells. Three to five areas in the bleached or unbleached half of the cell were selected for analysis. The intensity change of CFP was analysed using the Leica FRET AB Wizard software. The FRET efficiency was calculated using the following formula: statistical significance was determined using the Student’s t -test. As a control, we also made separate constructs of YFP-Sufu (YFP on the N terminus of Sufu) and Sufu–CFP (CFP on the C terminus of Sufu), transfected them together into HEK293T cells and performed FRET measurements to see whether there was a FRET signal between YFP and CFP tagged on different Sufu molecules. It is generally considered that the spatial proximity between YFP and CFP is not significant when the measured FRET efficiency is less than or close to 5%. Accession codes: The atomic coordinates and structure factors of FL hSufu, hSufuΔ60, hSufuΔ20, FL dSufu and the hSufuΔ60–hGli1 (112–128) complex have been deposited in the Protein Data Bank with accession numbers 4KM9 , 4KM8 , 4KMH , 4KMA and 4KMD , respectively. How to cite this article: Zhang, Y. et al. Structural insight into the mutual recognition and regulation between Suppressor of Fused and Gli/Ci. Nat. Commun. 4:2608 doi: 10.1038/ncomms3608 (2013).